Discovery and biosynthesis of karnamicins as angiotensin converting enzyme inhibitors Angiotensin-converting enzyme inhibitors are widely used for treatment of hypertension and related diseases. Here, six karnamicins E 1 -E 6 ( 1 – 6 ), which bear fully substituted hydroxypyridine and thiazole moieties are characterized from the rare actinobacterium Lechevalieria rhizosphaerae NEAU-A2. Through a combination of isotopic labeling, genome mining, and enzymatic characterization studies, the programmed assembly of the fully substituted hydroxypyridine moiety in karnamicin is proposed to be due to sequential operation of a hybrid polyketide synthase-nonribosomal peptide synthetase, two regioselective pyridine ring flavoprotein hydroxylases, and a methyltransferase. Based on AlphaFold protein structures predictions, molecular docking, and site-directed mutagenesis, we find that two pyridine hydroxylases deploy active site residues distinct from other flavoprotein monooxygenases to direct the chemo- and regioselective hydroxylation of the pyridine nucleus. Pleasingly, karnamicins show significant angiotensin-converting enzyme inhibitory activity with IC 50 values ranging from 0.24 to 5.81 μM, suggesting their potential use for the treatment of hypertension and related diseases. According to statistics from the World Health Organization (WHO), cardiovascular diseases (CVDs) are the leading cause of death globally, taking the lives of 17.9 million people in 2019. Perhaps more concerningly, 81% of these deaths occur in developing countries and over one third are defined as premature (i.e., 30–70 years of age) [1] . Hypertension, or elevated blood pressure, has been well recognized as the key risk factor for almost all CVDs acquired during life [2] . Of particular relevance to current public health measures, recent studies have also revealed that the prevalence of hypertension and CVD is clinically relevant in patients with COVID-19 [3] , [4] , [5] . Angiotensin-converting enzyme (ACE), a zinc-dependent dipeptide carboxypeptidase, is responsible for elevating human blood pressure by catalyzing the production of potent vasoconstrictor angiotensin-II from inactive angiotensin-I, as well as the degradation of vasodilator bradykinin [6] , [7] . Inhibition of ACE is a modern therapeutic target in the treatment of hypertension and related CVDs [8] , [9] . However, the widely used ACE inhibitors, such as captopril and enalapril, have relatively high incidence of side effects [10] , [11] , [12] , hindering their broad clinical application. Considering the potential of microbial natural products in drug discovery [13] , mining natural ACE inhibitor candidates from microorganisms is a promising approach. Pyridine, thiazole, and their bi-heteroaryl derivatives are common functionalities present in many clinically applied drugs, such as antihistamine brompheniramine, and anticancer agents ixabepilone and alpelisib [14] , [15] , [16] , [17] , [18] , [19] (Fig. 1a ). Notably, such moieties also form the core structure of the karnamicin natural products, a class of antibiotics originally isolated from the fermentation liquor of an actinobacterium, Saccharothrix aerocolonigenes N806-4, in 1989 [20] . Although only weak antibacterial activity was found against Gram-positive bacteria [20] , the unique skeleton composed of fully substituted hydroxypyridine and thiazole moieties indicates that there could be a wealth of potential bioactivities. However, other than the total synthesis of karnamicin B 1 achieved in 1997 [21] , no further studies of these compounds have been carried out. Exploring the karnamicin biosynthetic assembly line and analyzing their biological activities (other than antimicrobial) will help broaden and deepen our understanding of the medicinal potential of thiazole pyridine hybrid compounds, and further develop clinically important drugs. Fig. 1: Structures of brompheniramine, ixabepilone, alpelisib, and 1–7 and organization of related genes in the cae and knm BGCs. a Pharmaceuticals containing thiazole and/or pyridine ring. b Structures of karnamicins 1 – 7 , key COSY and HMBC correlations of 1 , ORTEP representation (30% probability ellipsoids) of the X-ray structure of compound 7 , and isotope labeling result. c Comparison of the organization of the cae BGC from A. cyanogriseus strain NRRL B-2194 and knm BGC from L. rhizosphaerae NEAU-A2. Full size image In this study, six karnamicins E 1 –E 6 ( 1 – 6 ), together with five known karnamicins ( 7 – 11 ) are isolated from Lechevalieria rhizosphaerae NEAU-A2 (Fig. 1b ), a rare actinobacterium isolated from rhizosphere soil of wheat ( Triticum aestivum ). Using 13 C-labeled precursor feeding, genome sequencing, and in vivo gene knockout and in vitro enzyme activity assays, we here dissect the biosynthetic gene cluster (BGC) responsible for assembling karnamicins in L. rhizosphaerae NEAU-A2 ( knm , Fig. 1c ). Interestingly, an unusual hybrid polyketide synthase-nonribosomal peptide synthetase (PKS-NRPS) KnmA2 is found to cooperate with two flavoprotein monooxygenases (FPMOs) KnmB1 and KnmB2, and a methyltransferase KnmF for assembling the characteristic fully substituted hydroxypyridine core in karnamicins. Subsequent structure-function relationship analysis demonstrates that, although KnmB1 and KnmB2 behave like other known aromatic hydroxylases, phylogenetically distinct active-site residues are recruited to realize the regioselective hydroxylation of the pyridine system. Finally, strong ACE inhibitory activity is established for a range of karnamicins, including less substituted biosynthetic intermediates, highlighting the potential of karnamicins as drug leads for hypertension and related CVDs. Discovery and structural elucidation of karnamicins E 1 –E 6 from L. rhizosphaerae NEAU-A2 Karnamicin E 1 ( 1 ) was obtained as colorless amorphous powder, and its molecular formula C 18 H 25 N 3 O 4 S was determined by high-resolution electrospray ionization mass spectrometry (HRESIMS) data ( m/z 380.1648 [M + H] + , Supplementary Fig. 1 ), corresponding to eight degrees of unsaturation. 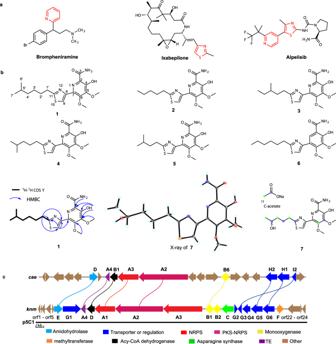Fig. 1: Structures of brompheniramine, ixabepilone, alpelisib, and 1–7 and organization of related genes in thecaeandknmBGCs. aPharmaceuticals containing thiazole and/or pyridine ring.bStructures of karnamicins1–7, key COSY and HMBC correlations of1, ORTEP representation (30% probability ellipsoids) of the X-ray structure of compound7, and isotope labeling result.cComparison of the organization of thecaeBGC fromA. cyanogriseusstrain NRRL B-2194 andknmBGC fromL. rhizosphaeraeNEAU-A2. The 1 H NMR spectrum and 13 C NMR and HSQC spectra showed the resonances of 18 carbons, which were classified into eight aromatic quaternary carbons, one carbonyl carbon, four sp 3 methylene carbons, one sp 3 methine carbon, two methyl carbons, and two methoxy carbons (Supplementary Table 1 and Supplementary Figs. 2 – 5 ). 1 H– 1 H correlation spectroscopy indicated the presence of one spin-coupling system, H-1′/H-2′/H-3′/H-4′/H-5′/H-6′(H-7′), as shown in Fig. 1b . Furthermore, the HMBC cross-peaks from O-Me-13 to C5, from O-Me-14 to C6, from NH to C2 and from OH-4 to C2/4/5 (Supplementary Fig. 6 ), revealed the presence of a 4-hydroxy-5,6-dimethoxy-pyridinecarboxamide moiety. Cross-peaks from H-9 to C-7/8/11 were observed in the HMBC spectrum (Supplementary Fig. 6 ), suggesting a 4-hydroxy-5,6-dimethoxy-7-thiazolyl-picolinamide moiety. Lastly, the 4-hydroxy-5,6-dimethoxy-7-thiazolyl-pyridinecarboxamide moiety and the alkyl chain were found to be attached at the C11 position, based on the key HMBC correlation from H-1′ to C11/C-9/C-8 (Fig. 1b ). It is noteworthy that the assignment of compound 1 was confounded by the lack of clear HMBC correlations, largely due to the high fraction of quaternary carbons and heteroatoms. Fortunately, however, the crystal structure of the also isolated compound 7 enabled unambiguous structural confirmation of the karnamicins by analogy (Fig. 1b ). The 1 H and 13 C NMR spectra of co-isolated 2 – 6 also showed high similarity to those of 1 and 7 , except for alkyl side chain substitutions (Fig. 1b ). Their structures were then determined based on extensive analyses of spectroscopic data (Supplementary Tables 2 – 6 and Supplementary Figs. 7 – 37 ). Identification of the karnamicin biosynthetic gene cluster Encouraged by their unique structural features, we set out to dissect the molecular basis for the biosynthetic assembly of karnamicins. Initially, an isotopic feeding study was conducted with L. rhizosphaerae NEAU-A2 using sodium [1- 13 C] and [2- 13 C] acetate and then spectrally analyzing the major product 7 . Treatment with [1- 13 C] acetate contributed to the enrichment in carbons C11, C5, C4′, and C2′ (Supplementary Fig. 38 ), while the 13 C signals derived from [2- 13 C] acetate were found to be distributed among carbons C6, C1′, C3′, and C5′ (Supplementary Fig. 39 ), suggesting intact incorporation of one acetate unit into the pyridine ring moiety (C5 to C6) and head-to-tail incorporation of three acetate units into the alkyl chain and thiazole ring (C5′ to C1′ and C11, Fig. 1b ). Further evidence supporting incorporation of intact acetate into the pyridine ring moiety was obtained by feeding [1, 2- 13 C 2 ] acetate (Supplementary Fig. 40 ). The presence of the acetate unit in the pyridine ring strongly suggested that a PKS participates in pyridine ring construction in karnamicin biosynthetic pathway. To gain further insight into the biosynthetic mechanism of the karnamicins, the genome of L. rhizosphaerae NEAU-A2 was sequenced and annotated using the prokaryotic genome annotation pipeline (GeneMarkS Version 2.0) [22] . Subsequent antiSMASH 4.0- [23] and PRISM 3-based [24] genome mining allowed the discovery of a potential BGC ( knm ) for synthesizing karnamicin in L. rhizosphaerae NEAU-A2. The knm BGC consisted of 16 open reading frames (ORFs), encoding proteins homologous to amidohydrolase (KnmE), transporters or regulators (KnmG1-KnmG6), thioesterase (TE, KnmA4), acyl-CoA dehydrogenase (KnmD), NRPSs (KnmA1 and KnmA3), PKS-NRPS (KnmA2), flavin adenine dinucleotide (FAD)-dependent monooxygenases (KnmB1 and KnmB2), asparagine synthase (KnmC), and methyltransferase (KnmF) (Fig. 1c and Supplementary Table 7 ). Intriguingly, gene cluster highly similar to the knm BGC was recognized in the genome of Actinoalloteichus cyanogriseus ( cae , GenBank NO. JQ687072) (Fig. 1c ), and moreover, cae BGC has been well established for biosynthesizing 2,2′-bipyridine antibiotics caerulomycin [25] , [26] . To examine the involvement of knm BGC in assembling the karnamicins, we first chose to inactivate the putative PKS-NRPS hybrid gene knmA2 in the cluster, whose homologs caeA2 and colA2 in cae and col clusters have been demonstrated to be responsible for constructing pyridine ring in caerulomycin and collismycin biosynthesis, respectively [25] , [26] , [27] . Based on the gene knockout system we developed in L . rhizosphaerae NEAU-A2 [28] , [29] , a Δ knmA2 mutant was obtained by homologous recombination (Supplementary Fig. 41 ). As expected, Δ knmA2 completely abolished the production of the karnamicins (Fig. 2 , trace vii), providing initial evidence supporting the relevance of the knm cluster in biosynthesizing karnamicin. Further single gene deletion experiments were then performed for knmA1 , knmB1 , knmB2 , knmC , knmE , and knmF in the cluster (Supplementary Fig. 41 ), with the altered (or absent) metabolite profile in the corresponding mutants (Fig. 2 ) confirming that the knm BGC was required for karnamicin assembly. Meanwhile, heterologous expression of knm BGC (cosmid p5C1, Fig. 1c ) in Streptomyces albus J1074 was carried out. Successful detection of karnamicins in the engineered strain S. albus 5C1 instead of the S. albus J1074 control (strain containing vector alone) further confirmed the dedicated role of knm BGC in synthesizing karnamicins (Fig. 2 , trace ii and Supplementary Fig. 42 , trace iii and iv). Notably, we found that the fatty acid side chain of karnamicins produced by S. albus 5C1 was not oxidized, indicating the lack of specific fatty acid oxidase in the heterologous host S. albus J1074. Fig. 2: HPLC analysis of metabolic extracts from wild-type L. rhizosphaerae NEAU-A2 (i, magnified region focuses on 1 – 6 ), heterologous expression strain S. albus 5C1 (ii) and mutant strains (iii-ix). Source data are provided as a Source Data file. Full size image Functional characterization of pyridine tailoring enzymes in knm BGC KnmA3 is a potential NRPS showing the greatest similarity to EpoB ( Sorangium cellulosum ) that assembles the thiazole ring in epothilone biosynthesis [30] , [31] , [32] (Supplementary Table 7 ). Meanwhile, KnmA1, KnmA2, KnmA4, and KnmD strongly resemble CaeA3, CaeA2, CaeA4, and CaeB1 involved in generating pyridine unit in caerulomycin biosynthesis [25] , [26] (Supplementary Table 7 ). Therefore, we instead sought to focus on potential post-tailoring enzymes for the targeted modification of the pyridine ring. Candidate enzymes based on gene annotations included a metal-dependent amidohydrolase (KnmE), two putative FAD-dependent monooxygenases (KnmB1 and KnmB2), asparagine synthase (KnmC), and methyltransferase (KnmF). We individually inactivated these enzyme genes in the heterologous host strain S. albus 5C1 using λ red-mediated PCR targeting mutagenesis [33] (Supplementary Fig. 43 ). However, only the S. albus 5C1-Δ knmB2 mutant was observed to accumulate presumable intermediates ( 24 – 26 and 32 – 33 , Fig. 2 , trace v), and therefore we chose to conduct further gene inactivation in wild-type strain L. rhizosphaerae NEAU-A2. KnmE, the putative metal-dependent amidohydrolase, showed the highest identity with CaeD from A. cyanogriseus NRRL B-2194 [34] (Supplementary Table 7 ). Interestingly, the Δ knmE strain retained the ability to produce karnamicins, while the accumulation of other metabolites was also observed ( 20 – 22 , Fig. 2 , trace ix). NMR and HRESIMS (Supplementary Figs. 37 , 44 – 61 and Supplementary Tables 8 – 10 ) analysis determined that compounds 20 – 22 are presumed karnamicin biosynthesis intermediates tailored with a l -leucine residue on C3 (Fig. 3 ). Given the absence of a leucine group on C3 of final karnamicin products, we proposed that KnmE was responsible for removing the l -leucine residue of intermediates 20 – 22 to afford the supposed intermediate 23 (Fig. 3 ). Moreover, since the formation of the target products karnamicins could be detected along with the accumulation of the intermediates 20 – 22 in the Δ knmE strain, it could be concluded that other amidohydrolases could also perform this catalysis, though they may not be as efficient as KnmE. KnmC was a predicted asparagine synthase that could be involved in the transamination of 23 (Fig. 3 ). We then inactivated knmC in the wild-type L. rhizosphaerae NEAU-A2 strain (Supplementary Fig. 41 ). The resultant mutant Δ knmC did not produce the karnamicins, nor its putative substrate 23 or other products (Fig. 2 , trace iv). Meanwhile, the gene complementation mutant S. albus 5C1-Δ knmC / knmC restored karnamicin production (Supplementary Fig. 42 ). Fig. 3: Proposed biosynthetic pathway for karnamicins. FAALs fatty acyl-AMP ligases, ACP acyl carrier protein, Cy condensation/cyclization domain, A adenylation domain, Ox flavin-dependent oxidase domain, PCP peptidyl carrier protein, KS ketosynthase, AT acyl transferase, C condensation domain, Ct terminal condensation domain, TE thioesterase. Full size image Bioinformatics analysis revealed that KnmB1 and KnmB2 resemble various group A FPMOs containing one Rossmann fold domain (GxGxxG signature) involved in FAD binding, one FAD-NAD(P)H binding motif (DG fingerprint), and one GD motif involved in contacting the riboflavin moiety of FAD [35] , [36] , [37] , [38] (Supplementary Table 7 and Supplementary Fig. 62 ). We thus hypothesized that KnmB1 and KnmB2 may be responsible for the hydroxylation of the pyridine core. Inactivation of knmB1 or knmB2 in the wild-type L. rhizosphaerae NEAU-A2 strain was then performed by PCR-targeted insertional mutation [29] , [33] (Supplementary Fig. 41 ). As expected, karnamicin production was not observed in either Δ knmB1 or Δ knmB2 mutant strains. Instead, we noticed the presence of the major products 36 and 37 , and a small amount of 35 in the Δ knmB1 mutant strain (Fig. 2 , trace vi), as well as major products 24–26 and minor products 32 and 33 in the Δ knmB2 mutant strain (Fig. 2 , trace v). NMR and HRESIMS-based structure elucidation (Supplementary Figs. 37 , 63 – 110 and Supplementary Tables 11 – 18 ) indicated that compounds 35–37 found in the Δ knmB1 strain possess an additional hydroxyl group on the pyridine core compared to 32–33 found in the Δ knmB2 mutant, while 32 and 33 were potential O -methylated derivatives of 24 and 26 , thus supporting the possible assembly logic that KnmB2 and KnmB1 were employed for the C4- and C6-hydroxylation of the pyridine core (Fig. 3 ), respectively. Notably, substrate promiscuity of the assembly line methyltransferase (likely KnmF) resulted in C5- O -methylation of the corresponding pyridine monohydroxylated or dihydroxylated intermediates 24–27 , yielding the methylated compounds 32–33 and 35 – 37 (Fig. 3 ) observed in the Δ knmB2 or Δ knmB1 mutant strains. To test the hypothesized role of KnmF, we chose to delete the knmF gene in-frame to avoid potential polar effects on the expression of downstream genes [33] (Supplementary Fig. 41 ). However, HPLC analysis of the culture extract of the Δ knmF mutant strain did not show the expected C5 or C6 demethylated products, or other karnamicin analogues (Fig. 2 , trace iii), which may be due to the instability of the trihydroxypyridine core of intermediate 28 (Fig. 3 ). In vitro characterization of hydroxylation and methylation at the pyridine core To further examine the catalytic role of methyltransferase KnmF and monooxygenases KnmB1 and KnmB2 during the karnamicin assembly process, we decided to characterize their enzyme activities in vitro. For KnmF, we synthesized 28 (Fig. 3 , Supplementary Figs. 111 – 116 , and Supplementary Table 19 ), a putative dedicated substrate of KnmF with a trihydroxypyridine core. Subsequently, a time course analysis of the enzyme-catalyzed reaction was performed with KnmF expressed by Escherichia coli BL21 (DE3) cells (Supplementary Fig. 117 ) and 28 . Intriguingly, immediately following the consumption of 28 , a compound 30 appeared. The subsequent decrease in abundance of 30 was accompanied by the accumulation of karnamicin E 1 ( 1 ) (Fig. 4a ). The structure of 30 was established by HRESIMS (C 17 H 24 N 3 O 4 S, m/z [M + H] + 366.1477, Supplementary Fig. 118 ) and NMR analyses (Supplementary Figs. 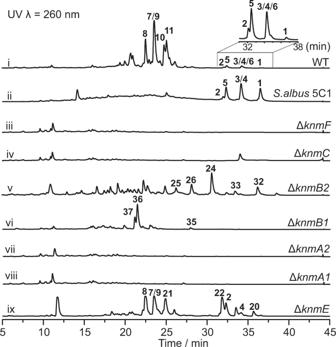Fig. 2: HPLC analysis of metabolic extracts from wild-typeL. rhizosphaeraeNEAU-A2 (i, magnified region focuses on1–6), heterologous expression strainS. albus5C1 (ii) and mutant strains (iii-ix). Source data are provided as a Source Data file. 37 , 119 – 123 and Supplementary Table 20 ). In addition, we also observed that synthetic 28 was degraded rapidly in the reaction buffer. Consequently, it was suggested that methyltransferase KnmF catalyzed the C5- O -methylation of 28 to afford 30 , followed by C6- O -methylation to give karnamicin E 1 ( 1 ) (Fig. 3 ). Fig. 4: HPLC analysis of the reactions catalyzed by KnmF, KnmB1, and KnmB2. a HPLC analysis of KnmF-catalyzed reactions in the presence of 28 , SAM and KnmF. (i) 2 h; (ii) 30 min; (iii) 15 min; (iv) the control reaction in the presence of 28 and SAM; (v) standard 1 . b HPLC analysis of KnmB1- and KnmB2-catalyzed reactions. (i) the control reaction in the presence of 24 , SAM and NADPH; (ii) the reaction in the presence of 24 , SAM, NADPH, KnmB2 and KnmF; (iii) the reaction in the presence of 24 , SAM and KnmF; (iv) the reaction in the presence of 24 , SAM, NADPH, KnmF, KnmB1 and KnmB2; (v) the reaction in the presence of 24 , NADPH, KnmB1 and KnmB2; (vi) standard 32 ; (vii) standard 30 ; (viii) standard 1 . Source data are provided as a Source Data file. Full size image The purified KnmB1 and KnmB2 proteins expressed in E. coli BL21(DE3) cells (Supplementary Fig. 117 ) were light yellow and released FAD upon boiling (Supplementary Fig. 124 ). Incubation of KnmB2 with 24 , the major product isolated from the Δ knmB2 mutant strain, did not generate any detectable product in the presence of the cofactors FAD and NAD(P)H, while the amount of 24 was reduced (Supplementary Fig. 125a , trace vi). Considering the accumulation of intermediates 35 – 37 with a C5- O -methylated instead of 4,5-dihydroxylated pyridine ring in the Δ knmB1 mutant strain, we speculated that the KnmB2-catalyzed hydroxylation product may be unstable, and that additional methyltransferase activity could stabilize the product through the O -methylation reaction. Consequently, we then investigated the catalytic reaction by incubating KnmB2 with 24 or 25 in the presence of the identified methyltransferase KnmF (Supplementary Fig. 125 ). In the event, HPLC analysis showed the conversion of 24 into two products 32 and 38 (Fig. 4b , trace ii). Based on the molecular formulas of 24 , 32 , and 38 (Supplementary Fig. 126 ), we proposed that 32 was the methylation product of 24 , and 38 was the methylation and oxidation product. Since KnmB2 could not catalyze conversion of 32 to 38 (Supplementary Fig. 125a , trace ii), this indicated that the C5-hydroxyl group of the pyridine core is necessary for KnmB2 activity. Overall, these findings indicated that KnmB2 selectively catalyzes the C4-hydroxylation of the pyridine ring. Investigation of the function of the likely hydroxylase KnmB1 in vitro was initially carried out by incubating the enzyme with 36 , the major product isolated from the Δ knmB1 mutant strain (Fig. 2 , trace vi). However, neither formation of products nor consumption of substrate was observed in the presence of NADPH (Supplementary Fig. 127a ), suggesting that KnmB1 was incapable of hydroxylating 36 at C6. In several previous examples, FPMO-catalyzed hydroxylation of aromatic rings is stimulated by deprotonation of an unmodified hydroxyl group ortho or para to the target position and the subsequent electrophilic attack by the reactive flavin C4a-hydroperoxide intermediate [38] , [39] , [40] . KnmB1 may behave in a similar way, meaning that C6-hydroxylation would proceed prior to the O -methylation of the C5-hydroxyl group. Accordingly, we set about preparing demethylated precursor 27 as a substrate for KnmB1 (Fig. 3 ). Unfortunately, attempts to obtain 27 by chemically demethylating 36 or 37 failed. Therefore, we chose to incubate 24 with KnmB1 in the presence of KnmB2 and KnmF to test the role of KnmB1. By HPLC analysis, the production of karnamicin E 1 ( 1 ) and monomethylated intermediate 30 was observed (Fig. 4b , trace iv). 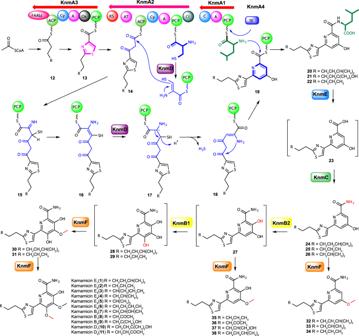Fig. 3: Proposed biosynthetic pathway for karnamicins. FAALs fatty acyl-AMP ligases, ACP acyl carrier protein, Cy condensation/cyclization domain, A adenylation domain, Ox flavin-dependent oxidase domain, PCP peptidyl carrier protein, KS ketosynthase, AT acyl transferase, C condensation domain, Ct terminal condensation domain, TE thioesterase. However, due to the instability of the trihydroxypyridine core, the putative enzymatic reaction product 28 was not observed when incubating 24 with KnmB1 and KnmB2 (Fig. 4b , trace v), which was in agreement with our observation that synthetic 28 was degraded rapidly in the reaction buffer. Altogether, these results highlight a biosynthetic procedure in which following the KnmB2-catalyzed C4-hydroxylation of 24 , KnmB1 activity completed the C6-hydroxylation of the pyridine core, and then KnmF was responsible for successive methylations of the C5- and C6-hydroxyl groups of 28 to yield karnamicin E 1 ( 1 ) (Fig. 3 ). Consistent with this procedure, in the presence of KnmF, 28 and 30 were completely converted into 1 within 2 h, while the transformation of 24 into 32 took more than 24 h. This also explains why the main product of the Δ knmB2 mutant was intermediate 24 rather than methylated product 32 . Catalytic mechanism of regioselective hydroxylases KnmB1 and KnmB2 In order to further understand the functional mechanism of regioselective hydroxylases KnmB1 and KnmB2, multiple sequence alignment and phylogenetic analyses of KnmB1, KnmB2, and other reported FPMOs responsible for hydroxylation of pyridine nucleus or aromatic rings were performed (Supplementary Figs. 62 and 128 ). It was established that KnmB1 and KnmB2 belong to group A FPMOs [41] with the characteristic conserved FAD binding sites [35] (GXGXXG…DG…GD, Supplementary Fig. 62 ). KnmB1 showed the highest sequence identity with CaeB6 (55%), a selective hydroxylase in the biosynthesis of the 2,2ʹ-bipyridine compounds caerulomycins [40] , and 2-methyl-3-hydroxypyridine-5-carboxylic acid oxygenase (MHPCO, 45%), an enzyme catalyzing the oxidative pyridine ring-opening reaction of vitamin B6 degradative pathway in Mesorhizobium loti MAFF303099 [42] . Although only 30.6% of the amino acid sequence identity was elucidated, the enzyme most similar to KnmB2 was found to be HpxO, a flavin-dependent urate oxidase that catalyzes the hydroxylation of uric acid to yield a 5-hydroxyisourate intermediate of a purine catabolic pathway in Klebsiella pneumoniae [43] . Among these enzymes, crystal structures and catalytic mechanisms of MHPCO and HpxO have been investigated [42] , [43] . However, the conserved catalytic residues elucidated in MHPCO/HpxO could not be identified in KnmB1/KnmB2 by amino acid sequence alignments (Supplementary Fig. 62 ). We hypothesized that distinct active-site architecture may be employed by KnmB1/B2 for hydroxylation of the pyridine nucleus. Despite many attempts, we were unable to obtain crystals of the KnmB1 or KnmB2 protein suitable for X-ray crystallographic analysis. Fortunately, the recent success of AlphaFold has demonstrated the values of artificial intelligence (AI) methods in predicting highly accurate protein structures, which we chose to deploy in this setting [44] . Interestingly, the overall structure of KnmB1 or KnmB2 predicted by AlphaFold was highly similar to that of PHBH (Fig. 5a ) and other flavoprotein aromatic hydroxylases [41] , thus raising the question of whether KnmB1 and KnmB2 acomplish the pyridine ring hydroxyation in a way similar to that of the reported aromatic ring hydroxylases. To unravel the structure-function relationship of KnmB1 and KnmB2, we performed a molecular docking analysis using the predicted protein structures and their corresponding substrates ( 27 for KnmB1, and 24 for KnmB2). As shown in Fig. 5 , potential hydrogen bond interactions between substrate 27 , especially its amide and hydroxyl groups, and residues Asn219, Tyr262, Arg205, and Tyr217, in KnmB1 were present (Fig. 5b ). For KnmB2, the residues Asn291 and Tyr215 were predicted to form hydrogen bonds with substrate 24 , while Phe205 was suggested to exhibit π-π stacking interaction with the pyridine ring (Fig. 5c ). Particularly, the side chains of Asn219/291 and Tyr217/215 in KnmB1 and KnmB2 were predicted to be hydrogen bond donors, which may act by deprotonating substrate for oxygen activation. While the active sites of KnmB1 and KnmB2 do bear some homology to other flavoprotein aromatic hydroxylases and group A FPMOs (MHPCO [42] and HpxO [43] also utilize tyrosine in forming hydrogen bond with their respective substrates), other residues, such as Asn219 and Tyr262 in KnmB1 and Asn291 and Phe205 in KnmB2, are notably unique. Fig. 5: Structures and catalytic mechanisms of KnmB1 and KnmB2. a Comparison of the overall structures of KnmB1 (green), KnmB2 (cyan), and p -hydroxybenzoate hydroxylase (PHBH; pdb:1pbe; pink). b Molecular docking of 27 in KnmB1. c Molecular docking of 24 in KnmB2. N, O, and S atoms are colored blue, red and yellow, respectively. C atoms in KnmB1 residues, KnmB2 residues, and small molecules are colored as green, cyan, and white, respectively. d Proposed catalytic mechanism of KnmB1. e Proposed catalytic mechanism of KnmB2. R is ribityl adenosine diphosphate for FAD. Full size image To test the role of these predictive active-site residues in determining the catalytic activity of KnmB1/B2, a series of site-directed mutants of KnmB1 (N219D, Y217A/F, Y262A and R205A) and KnmB2 (N291D, Y215A/F and F205A) were respectively generated. In comparison with wild-type, ~26–70% decrease in FAD content was observed in all enzyme variants except the Y217A mutant of KnmB1 (Supplementary Fig. 129 ), indicating that the FAD binding is perturbed in these variants. Interestingly, in vitro enzymatic assays revealed that these enzyme mutants lost all hydroxylation activity towards 27 or 24 (Supplementary Fig. 130 ). However, the possibility that site-directed mutations may have led to gross changes in tertiary protein structure, which would also lead to a substantial loss of FAD binding and catalytic activity, could be ruled out, since these variants retained the NADPH oxidase activity observed in wild-type enzymes (Supplementary Fig. 131a–c ). Inspired by this result, we chose to explore the catalytic features of KnmB1 and KnmB2 by monitoring the kinetics of NADPH consumption and hydrogen peroxide (H 2 O 2 ) formation in time. First, it is interesting to note that, KnmB1 and particularly KnmB2 have noticeable NADPH oxidase activity regardless of the presence of a hydroxylatable ( 24 for KnmB2, coupling efficiency 0–45%) or non-hydroxylatable ( 24 for KnmB1, and 32 for KnmB2) effector (Supplementary Fig. 131d–j ), suggesting that these two group A FPMOs are inefficient at inhibiting wasteful flavin reduction in the absence of any effector. Second, as a non-deprotonatable ligand, methylated product 32 could dramatically stimulate the reaction of KnmB2 with NADPH, even to a greater extent than that the substrate 24 did (Supplementary Fig. 131i , j). This means that features other than an activating substituent on the pyridine ring were sensed and triggered rapid acceleration of flavin reduction in KnmB2. For KnmB1, its direct substrate 27 is not available. However, 24 but not 32 or 36 could act as a non-substrate effector to accelerate the reduction of flavin in KnmB1 by NADPH (Supplementary Fig. 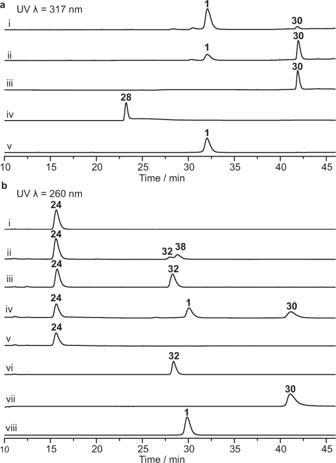Fig. 4: HPLC analysis of the reactions catalyzed by KnmF, KnmB1, and KnmB2. aHPLC analysis of KnmF-catalyzed reactions in the presence of28, SAM and KnmF. (i) 2 h; (ii) 30 min; (iii) 15 min; (iv) the control reaction in the presence of28and SAM; (v) standard1.bHPLC analysis of KnmB1- and KnmB2-catalyzed reactions. (i) the control reaction in the presence of24, SAM and NADPH; (ii) the reaction in the presence of24, SAM, NADPH, KnmB2 and KnmF; (iii) the reaction in the presence of24, SAM and KnmF; (iv) the reaction in the presence of24, SAM, NADPH, KnmF, KnmB1 and KnmB2; (v) the reaction in the presence of24, NADPH, KnmB1 and KnmB2; (vi) standard32; (vii) standard30; (viii) standard1. Source data are provided as a Source Data file. 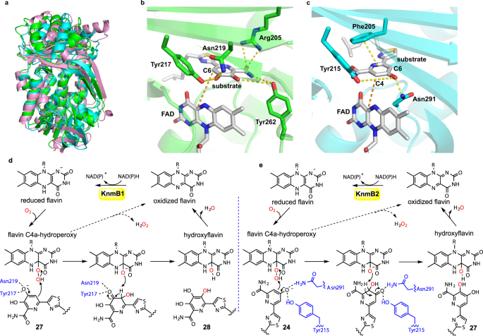Fig. 5: Structures and catalytic mechanisms of KnmB1 and KnmB2. aComparison of the overall structures of KnmB1 (green), KnmB2 (cyan), andp-hydroxybenzoate hydroxylase (PHBH; pdb:1pbe; pink).bMolecular docking of27in KnmB1.cMolecular docking of24in KnmB2. N, O, and S atoms are colored blue, red and yellow, respectively. C atoms in KnmB1 residues, KnmB2 residues, and small molecules are colored as green, cyan, and white, respectively.dProposed catalytic mechanism of KnmB1.eProposed catalytic mechanism of KnmB2. R is ribityl adenosine diphosphate for FAD. 131f ), indicating that the deprotonatable C5-hydroxyl group of the ligand is specifically required for exerting effector function upon binding to KnmB1. Based on the established understanding of group A FPMO-catalyzed hydroxylation of aromatic compounds [45] , [46] , it is reasonable to infer that the side chains of residues such as Asn219/291 and Tyr217/215 likely participate in forming the critical hydrogen bond networks responsible for proton transfer in the catalytic cycle of KnmB1/2. The proton transfer system is suggested to be required for substrate deprotonation, which is an essential step to drive the conformational changes (“out” and “in”) of cofactor flavin for reduction by NADPH, and to activate the substrate for electrophilic attack by flavin C4a-hydroperoxide intermediate [47] . Therefore, mutation of KnmB1 at Asn219 (N219D) or Tyr217 (Y217A/F) resulted in complete loss of response to non-substrate effector 24 (Supplementary Fig. 131e–g ). Meanwhile, in agreement with the finding that accelerated flavin reduction in KnmB2 was independent of the presence of an activating substituent on the pyridine ring, the substrate effector role of 24 in promoting flavin reduction was retained (though decreased) in N291D or Y215F mutant of KnmB2 (Supplementary Fig. 131h–j ). Nevertheless, the two mutants lost all hydroxylation activity towards 24 , which is probably due to impaired electrophilic substitution in the oxidative half-reaction resulting from deficiency in substrate deprotonation. Notably, binding and the proper orientation of substrate in the active site, which may be attributed to the side chains of Tyr262/Arg205 (KnmB1) and Phe205 (KnmB2), is also decisive for the reaction. Mutation in any of these residues resulted in a reduced (Y262A) or absent (R205A and F205A) response of KnmB1/2 to their effectors (Supplementary Fig. 131g, i ). In addition, different from Y215F mutant, large-to-small amino acid substitution at Tyr215 in KnmB2 (Y215A) led to loss of response to substrate 24 (Supplementary Fig. 131i ), which may be ascribed to improper binding or positioning of the substrate owing to steric change of the active-site cavity. Based on these results, a possible catalytic mechanism for the KnmB1- and KnmB2-catalyzed hydroxylation of the pyridine ring in karnamicin biosynthesis was proposed (Fig. 5 d, e ), which is analogous to that of group A FPMOs employing a flavin C4a-hydroperoxide intermediate [48] . More importantly, though, these structural studies suggest that KnmB1 and KnmB2 facilitate the chemo- and regiospecific hydroxylation of the pyridine nucleus through the exquisite arrangement of the enzyme-specific active-site residues, which are notably distinct from other FPMOs. This underlines the great diversity and unique regioselectivity of group A FPMOs [38] , [41] . Karnamicins as efficient ACE inhibitors Derivates of pyridines, thiazoles, and pyridine-thiazole hybrids have been well recognized as bioactive candidates with great potential for medical applications [14] , [15] , [16] , [17] , [18] , [19] . As a class of compounds with a unique skeleton composed of fully substituted hydroxypyridine and thiazole moieties, we first conducted a preliminary investigation of antibacterial and antifungal activities of karnamicins 1 – 11 against plant pathogens. However, only weak activity was found. Interestingly, in an attempt to explore natural ACE inhibitors for hypertension treatment, we surprisingly found that karnamicins isolated from wild-type and mutant strains had significant ACE inhibitory activity with IC 50 (the concentration yielding 50% inhibition) values ranging from 0.24 to 5.81 μM (except compound 32 , Table 1 ). Furthermore, analysis of the structure-activity relationship seems to imply that alkyl side chain hydroxylation leads to a two- to fivefold increase in activity. These activities bode well for future medicinal chemistry optimization, and point to the potential use of karnamicin derivatives as a treatment for hypertension. Table 1 ACE inhibitory activity a of karnamicins Full size table In this study, we presented the isolation and structural elucidation of karnamicins 1 – 11 with a unique skeleton composed of fully substituted hydroxypyridine and thiazole moieties from L. rhizosphaerae NEAU-A2 (Fig. 1b ). On the basis of 13 C-labeled precursor feeding, genome sequencing, bioinformatic analysis, in vivo gene knockout, and heterogeneous expression, we determined that the karnamicin biosynthetic assembly line was encoded by an unreported BGC named as knm (Fig. 1c ). Among the deduced protein products of knm BGC, KnmA1, KnmA2, KnmA3, KnmA4, and KnmD, showed clear similarities to enzymes that have been identified to be involved in generation of thiazole ring and pyridine ring moieties [25] , [26] , [27] , [30] , [31] , [32] . Subsequent characterization of enzymes responsible for the post-modification of the pyridine moiety led to the final elucidation of the complete biosynthetic pathway for karnamicins (Fig. 3 ). Quite recently, enzymes showing high similarity to PKS/NRPS hybrid protein KnmA2 and the acyl-CoA dehydrogenase KnmD (Supplementary Table 7 ) have been found to act synergistically to generate 2,2’-bipyridine in the caerulomycin (CaeA2 and CaeB1) and collismycin (ColA2 and ColB1) biosynthetic assembly lines [26] . Therefore, we speculated here that KnmA2 and KnmD afforded the pyridine ring moiety in the karnamicins by the same mechanism. The domains of NRPS KnmA1 were organized as C-A-PCP for l -leucine extension of 19 , and with the help of thioesterase KnmA4, the corresponding products 20 – 22 were released. Subsequently, KnmE removed the l -leucine residue to afford intermediate 23 . KnmC activity was required for the transamination reaction to yield 24–26 . Then, KnmB2-catalyzed hydroxylation of C4 affording dihydroxylated pyridine intermediate 27 , which was further oxidized by KnmB1 to form the trihydroxypyridine core of 28 . Finally, the karnamicin assembly was completed by successive KnmF-catalyzed O -methylation of 28 (Fig. 3 ). Intriguingly, genome mining using knm BGC as bait further resulted in the identification of another putative karnamicin-producing cluster from L. aerocolonigenes NBRC 13195 ( knmH , GenBank No. GCA_000974445.1, Supplementary Fig. 132 ), providing additional resources for karnamicin production. FPMOs are a class of enzymes that are capable of catalyzing a diverse set of chemo-, regio-, and enantio-selective oxyfunctionalization reactions [41] . In the knm BGC, KnmB2 and KnmB1 were identified as two FPMOs responsible for regioselective hydroxylation of the pyridine core, contributing substantially to the formation of the unique skeleton composed of fully substituted hydroxypyridine and thiazole moieties in the karnamicins. In agreement with this specific catalytic activity, amino acid sequence alignment, AlphaFold-based protein structure prediction, and site-directed mutations demonstrated that KnmB2/B1 recruited active sites distinct from other known aromatic ring hydroxylases to accomplish the hydroxylation of the pyridine nucleus, broadening our understanding of the diverse origin and functional evolution of pyridine hydroxylases in the FPMOs family. Consequently, the characterization of KnmB2/B1 provided important insights into the development of pyridine hydroxylase variants with designer properties for the production of pharmaceutical ingredients and fine chemicals. This is all the more important given the significant ACE inhibitory activity of the karnamicins, which could be used for the development of natural product-derived antihypertensive agents. General experimental procedures General materials and reagents used in this study are summarized in Supplementary Information. The bacterial strains, plasmids, and primers used in this study are summarized in Supplementary Tables 21 – 23 . Chromaster was used for HPLC data collection. MEGA version 7 was used for amino acid alignment and phylogenetic tree construction. OriginPro 9.0 was used for data visualization. MestReNova 6.1 was used for NMR data analysis. ChemBioDraw Ultra 20.0 was used for drawing chemical structures (Figs. 1 – 3 ). GeneMarkS Version 2.0 [22] was used for the prokaryotic genome annotation. antiSMASH 4.0 [23] and PRISM 3 [24] were used for genome mining. The sequence alignment of gene clusters was created using Clustal Omega and the figure was produced using EsPript 3.0. Isolation and purification of 1–11 from L. rhizosphaerae NEAU-A2 L. rhizosphaerae NEAU-A2 was grown on ISP3 agar plates [28] (Oatmeal 2%, KNO 3 0.02%, MgSO 4 ·7H 2 O 0.02%, K 2 HPO 4 ·3H 2 O 0.05% and Agar 2%, w/v, pH 7.2) for 5 days at 30 °C. Then, the mycelium was inoculated into 250 mL baffled Erlenmeyer flasks containing 50 mL of seed medium (TSB, Tryptone Soy Broth, 30 g/L) and cultivated for 2 days at 30 °C on a rotary shaker (200 rpm). After that, 5% (v/v) of the seed culture was transferred into 1000 mL baffled Erlenmeyer flasks filled with 300 mL of production medium B consisting of 0.5% soluble starch (w/v), 0.2% tryptone (w/v), 1% glucose (w/v), 0.2% yeast extract (w/v), 0.4% NaCl (w/v), 0.05% K 2 HPO 4 ·3H 2 O (w/v), 0.05% MgSO 4 ·7H 2 O (w/v), and 0.2% CaCO 3 (w/v), and cultured on a rotary shaker (200 rpm) at 30 °C for a week. The fermentation broth (40 L) was centrifuged (3488× g , 20 min), and the supernatant was extracted with ethyl acetate thrice. The ethyl acetate extract was concentrated to afford 10.0 g of oily crude extract. The mycelia were extracted with methanol (1 L × 3) and then concentrated in vacuo to remove the methanol to yield the aqueous concentrate. This aqueous concentrate was finally extracted with ethyl acetate (1 L × 3) to give 1.0 g of oily crude extract. Finally, two parts of the extracts were combined for further purification. The crude extract in total (11.0 g) was applied to silica gel column chromatography using a successive elution of petroleum ether/ethyl acetate (1:0, 20:1, 10:1, 5:1, 3:1, 1:1, and 0:1, v/v) to yield fractions A–F. Fr. A (petroleum ether/ethyl acetate, 1:1, v/v) was subjected to semipreparative HPLC-DAD (0–40.0 min, 50% CH 3 CN in H 2 O; 40.1–60.0 min, 55% CH 3 CN in H 2 O; 60.1–70.0 min, 70% CH 3 CN in H 2 O) directly to afford 5 ( t R = 37.0 min, 5.0 mg), 2 ( t R = 39.2 min, 6 mg), and 6 ( t R = 55.0 min, 4.4 mg). Fr. A-52 min was further purified by semipreparative HPLC-DAD (CH 3 CN:H 2 O = 44:56, v/v) to give 3 (3.0 mg) and 4 (5.0 mg). Fr. A-67 min was also further separated using the same semipreparative HPLC-DAD (CH 3 OH:H 2 O = 80:20, v/v) to provide 1 ( t R = 32.6 min, 4.8 mg). Fr. D (ethyl acetate) was subjected to semipreparative HPLC (0–28.0 min, 35% CH 3 CN in H 2 O; 28.1–43.0 min, 40% CH 3 CN in H 2 O) to yield 7 ( t R = 26.0 min, 20 mg). Fr. D-31.7 min was further purified by semipreparative HPLC to give 9 (13 mg) and 8 (11.2 mg). Fr. D-41.3 min was further purified by means of semipreparative HPLC to yield 11 (7 mg). Fr. E was submitted to semipreparative HPLC (0–27.0 min, 35% CH 3 CN in H 2 O; 27.1–43.0 min, 40% CH 3 CN in H 2 O; 43.1–48.0 min, 100% CH 3 CN) to obtain 10 ( t R = 26.0 min, 11.0 mg). X-ray crystallographic analysis of compound 7 Crystal data for 7 : C 16 H 21 N 3 O 5 S, M = 367.42, a = 8.489(2) Å, b = 20.732(5) Å, c = 9.931(2) Å, α = 90°, β = 106.838(4)°, γ = 90°, V = 1672.9(7) Å 3 , T = 100(2) K, space group P 21, Z = 4, μ (MoKα) = 0.227 mm -1 , 17516 reflections measured, 8938 independent reflections ( R int = 0.0755). The final R 1 values were 0.0629 ( I > 2 σ ( I )). The final wR ( F 2 ) values were 0.1387 ( I > 2 σ ( I )). The final R 1 values were 0.1055 (all data). The final wR ( F 2 ) values were 0.1583 (all data). The goodness of fit on F 2 was 1.011. Flack parameter = 0.21(10). Isolation and purification of metabolites from the mutant strains Based on HPLC analysis results of the mutant cultures, we selected Δ knmE , Δ KnmB1 , and Δ KnmB2 mutants for large-scale fermentation (20 L) using the aforementioned method and medium. The metabolites of the mutant strains were isolated and purified by silica gel column chromatography combined with thin-layer chromatography and semipreparative RP-HPLC. Finally, 20 , 21 , and 22 were isolated from the mutant strain NEAU-A2-Δ knmE . 24 , 25 , 26 , 32 , and 33 were obtained from the mutant strain S. albus 5C1-Δ knmB2 . Compounds 35 , 36 , and 37 were separated from the mutant strain NEAU-A2-Δ knmB1 . Isotopic labeling experiments Three 13 C-labeled compounds, [1- 13 C] sodium acetate, [2- 13 C] sodium acetate, and [1, 2- 13 C 2 ] sodium acetate, were used for the feeding experiments. Briefly, three 13 C-labeled compounds (500 mg) were individually dissolved in ddH 2 O at a concentration of 250 mg/mL as stock solution. L. rhizosphaerae NEAU-A2 was grown in seed medium (TSB) for 30 h, and the resultant seed culture (5% inocula) was then inoculated into 500 mL production medium at 30 °C on a rotary shaker (220 rpm). After 12, 24, and 36 h of incubation, a 13 C-labeled precursor ([1- 13 C], [2- 13 C], or [1, 2- 13 C 2 ] sodium acetate) was added into culture with the volume of 0.5 mL, 1 mL, and 0.5 mL, respectively, fermented for additional 3 days. Then, the culture was harvested and extracted with ethyl acetate for three times. The extracts were subjected to semipreparative HPLC-DAD directly to afford isotopic labeling compound 7 using an isocratic elution of 35% (v/v) acetonitrile containing 0.1% (v/v) acetic acid with a flow rate of 3 mL/min. Genomic library construction DNA isolation and manipulation in L. rhizosphaerae NEAU-A2 were performed according to standard manufacturer’s protocol [33] . Genomic library of L. rhizosphaerae NEAU-A2 was constructed in SuperCos I and pJTU2554 by using the Gigapack III Gold Packaging Extract system according to the manufacturer’s instructions (Stratagene). Briefly, the genomic DNA was partially digested with Mbo I. Then, the 30–42 kb DNA fragments were isolated and ligated to cosmid pJTU2554 and pSuperCos I. MaxPlax Lambda packaging extracts were used to packaging. About 4000 E. coli clones were picked from cosmid pJTU2554 genomic library, and about 2000 E. coli clones were picked from cosmid SuperCos I genomic library. They were then stored in 96-well microplates at −80 °C. Heterologous expression and gene inactivation experiments The positive cosmid, p5C1 from cosmid pJTU2554 genomic library, was introduced to the selected model Streptomyces host ( S. albus J1074) by E. coli – Streptomyces conjugation to obtain strain S. albus 5C1 according to the standard protocol [33] . Cosmid p5C1 which contains the whole knm gene cluster was used for the construction of gene deletion mutant. The λ -Red-mediated gene replacements were carried out following standard procedures [33] , [49] using the primers listed in Supplementary Table 22 . Finally, five markerless gene inactivation mutants (Δ knmE , Δ knmB1 , Δ knmB2 , Δ knmC and Δ knmF ) were constructed in this study. The PCR verification of the mutants are shown in Supplementary Fig. 43 with corresponding primers listed in Supplementary Table 22 . The gene inactivation experiments were carried out in wild-type strain L. rhizosphaerae NEAU-A2. Briefly, apramycin resistance gene cassettes ( aac(3)IV-oriT surrounded by FRT sites ) with 39 bp homologous to each side of the gene to be inactivated were amplified from plasmid pIJ773 by PCR using the primers listed in Supplementary Table 22 . Each of the apramycin resistance gene cassette was then introduced by electroporation into E. coli BW25113/pIJ790/S4H1, BW25113/pIJ790/S20G3, or BW25113/pIJ790/S12G3. The correctly mutated cosmids were introduced into E. coli ET12567/pUZ8002 by electroporation and then transferred into L. rhizosphaerae NEAU-A2 through intergeneric conjugation. Exconjugants resistant to apramycin were randomly isolated and tested for the loss of kanamycin resistance. Further, double crossover mutant strains were confirmed by PCR using primers listed in Supplementary Table 22 . Finally, seven mutants (Δ knmE , Δ knmA1 , Δ knmA2 , Δ knmB1 , Δ knmB2 , Δ knmC and Δ knmF ) were successfully constructed in L. rhizosphaerae NEAU-A2. The PCR verification of the mutants are shown in Supplementary Fig. 41 . All mutants were cultivated in medium B for 5 days and the metabolic extracts were monitored by HPLC-DAD. The HPLC analysis was performed at a flow rate of 1 mL/min with DAD detection using a 45 min solvent gradient as follows: T = 0 min, 8% B; T = 32 min, 80% B; T = 36.1 min, 90% B; T = 40 min, 100% B; T = 40.1 min, 8% B; T = 45 min, 8% B (A, H 2 O; B, MeCN), and the column temperature was 25 °C (Analytical method A). Chemical synthesis of compound 28 To a solution of 1 (9 mg) in dichloromethane (2 mL) was added BBr 3 (500 µL) at −78 °C under N 2 atmosphere [50] . The reaction was stirred at −78 °C for 30 min and was then warmed up to rt. The reaction was then stirred at rt for 10 h. The reaction mixture was slowly added into 4 mL saturated NaHCO 3 solution at 0 °C. The aqueous layer was extracted by ethyl acetate for three times and the combined organic layers were purified using RP-HPLC to afford 28 (4.4 mg). In vitro assay of KnmB1, KnmB2, and KnmF The reaction of KnmF was carried out at 30 °C in a 100 µL system containing 50 mM Tris-HCl buffer (pH 7.5), 1 mM compound 28 , 2 mM SAM, and 2 μM KnmF. After 15 min, 30 min, and 2 h, an equal volume of MeOH was added to the assay to quench the reaction. After centrifugation (10 min at 13,523× g ), the supernatant was analyzed by HPLC-DAD with solvent gradient as follows: T = 0 min, 55% B; T = 13.5 min, 55% B; T = 19 min, 65% B; T = 35 min, 65% B; T = 40 min, 100% B; T = 45 min, 100% B; T = 45.1 min, 55% B; T = 51 min, 55% B (A, H 2 O + 0.1% CH 3 COOH, v/v; B, MeCN), and the column temperature was 25 °C (Analytical method B). The reaction of KnmB1 was carried out at 30 °C in a 100 µL system containing 50 mM Tris-HCl buffer (pH 7.5), 0.2 mM compound 36 , 1 mM NADPH, and 5 μM KnmB1. The reaction of KnmB2 and KnmF was carried out at 30 °C in a 100 µL system containing 50 mM Tris-HCl buffer (pH 7.5), 0.2 mM compound 24 or 25 , 1 mM NADPH (NADH), 1 mM SAM, 2 μM KnmF, and 5 μM KnmB2. The reaction of KnmB1, KnmB2, and KnmF was performed at 30 °C in a 100 µL system containing 50 mM Tris-HCl buffer (pH 7.5), 0.2 mM compound 24 , 2 mM NADPH (NADH), 1 mM SAM, 5 μM KnmB1, 5 μM KnmB2 and 2 μM KnmF. After 4 h, an equal volume of MeOH was added to the assay to quench the reaction. After centrifugation (10 min at 13,523× g ), the supernatant was analyzed by HPLC-DAD with a YMC-Triart C 18 column (250 mm × 4.6 mm i.d., 5 μm) at a flow rate of 1.0 mL/min, solvent gradient as follows: T = 0 min, 55% B; T = 13.5 min, 55% B; T = 19 min, 65% B; T = 48 min, 65% B; T = 48.1 min, 100% B; T = 53 min, 100% B; T = 53.1 min, 55% B; T = 58 min, 55% B (A, H 2 O + 0.1% CH 3 COOH, v/v; B, MeCN), and the column temperature was 25 °C (Analytical method C). Determination of the flavin cofactor of KnmB1 and KnmB2 The protein solutions of KnmB1 and KnmB2 were incubated at 100 °C for 10 min for denaturation. After centrifugation, the supernatants were subjected to HPLC-DAD analysis on a C 18 column eluted with a flow rate of 1 mL/min over a 28 min gradient as follows: T = 0 min, 10% B; T = 20 min, 100% B; T = 24 min, 100% B; T = 24.1 min, 10% B; T = 28 min, 10% B (A, H 2 O; B, CH 3 OH) (Analytical method D). Standard FAD was used as control. Molecular docking Molecular docking was performed using Autodock Vina 1.2.2 [51] . The ligand substrates 24 , 27 , and FAD were generated using ChemBio3D Ultra 12.0, and then energy minimized with Molecular Mechanics (MM2) until a minimum root-mean-square (RMS) gradient of 0.100 was performed ( https://www.chemdraw.com.cn/ ). Then, substrates 24 and 27 were docked into the binding pocket of protein KnmB1 and KnmB2 based on AlphaFold protein structures prediction. During docking, the critical parameters such as grid number and algorithm were set to default values, but rotatable bonds in the ligand were not set in this manner in order to allow for flexible docking. Finally, 100 independent docking runs were performed, and the complex structure with the best combination of low binding energy and favorable orientation was selected. The resulting poses were analyzed and checked for hydrogen bonding in the PyMOL 2.5.2 ( http://www.pymol.org ) Molecular Graphics System. Angiotensin-converting enzyme inhibitor of assay ACE inhibitory activities were evaluated according to literatures [52] , [53] , [54] . Test compounds were dissolved in DMSO (10 mM), then diluted to afford serial concentrations with 80 mM HEPES-300 mM NaCl buffer (HEPES-NaCl, pH 8.3). Each compound solution was incubated with ACE solution (0.02 U/mL in HEPES-NaCl buffer) at 37 °C for 10 min in the 96-well microtiter plate. Then, FAPGG (dissolved in HEPES-NaCl buffer) was added and fully mixed. The initial absorbance value of each well was immediately measured at 340 nm and recorded as A 0 . After incubating at 37 °C for 30 min, the absorbance value at the end of the reaction of each well was measured at 340 nm again and denoted as A 30 . The decrease in the 340 nm absorbance was expressed as \(\varDelta A={A}_{0}-{A}_{30}\) . The ACE inhibition (percent) was calculated as follows: 
    R(%)=(A_NC-A_S)/A_NC× 100
 (1) where Δ A NC is the absorbance value of negative control and Δ A S is the absorbance value of the sample to be tested. The percentages of ACE inhibition were plotted vs Log 10 inhibitor concentrations obtaining a sigmoid curve. The IC 50 values (50% ACE activity inhibition), were estimated with GraphPad Prism 7.0 sigmoidal dose-response plots of inhibitor concentration (μM) versus percent inhibition. Captopril was used as a positive control. The results represent the mean IC 50 value ± standard deviation of three independent assays. Reporting summary Further information on research design is available in the Nature Portfolio Reporting Summary linked to this article.